Localized cell stimulation by nitric oxide using a photoactive porous coordination polymer platform Functional cellular substrates for localized cell stimulation by small molecules provide an opportunity to control and monitor cell signalling networks chemically in time and space. However, despite improvements in the controlled delivery of bioactive compounds, the precise localization of gaseous biomolecules at the single-cell level remains challenging. Here we target nitric oxide, a crucial signalling molecule with site-specific and concentration-dependent activities, and we report a synthetic strategy for developing spatiotemporally controllable nitric oxide-releasing platforms based on photoactive porous coordination polymers. By organizing molecules with poor reactivity into polymer structures, we observe increased photoreactivity and adjustable release using light irradiation. We embed photoactive polymer crystals in a biocompatible matrix and achieve precisely controlled nitric oxide delivery at the cellular level via localized two-photon laser activation. The biological relevance of the exogenous nitric oxide produced by this strategy is evidenced by an intracellular change in calcium concentration, mediated by nitric oxide-responsive plasma membrane channel proteins. Controlled cell stimulation by gaseous bioactive molecules is appealing for investigating cellular mechanisms and signalling networks, and for developing new therapeutic approaches [1] , [2] . The design of functional scaffolds or devices that can release molecules with precisely controlled timing, dosage and location remains challenging, especially for gaseous molecules, due to handling issues that arise from their high reactivity and physical state. Nitric oxide (NO) is one of the most investigated gasotransmitters, having a large role in numerous signalling events, including proliferation and vasodilatation [3] , [4] . Moreover, microenvironmental modulation by endogenous NO is believed to affect both physiological conditions, such as synaptic transmission, and also tissues and cancer stem cells [5] , [6] . Great effort has recently gone into the design of controllable NO-releasing scaffolds; however, the precise localization of NO delivery at the cellular level has not yet been demonstrated. We focus on the development of functional cellular substrates that provide on-demand NO release at multiple, well-defined locations. Stable compounds that are able to produce NO through a photochemical reaction are a promising means of achieving temporal control over NO release, and a variety of NO photodonors have been recently developed [7] , [8] , [9] . Light provides a noninvasive trigger, which can be highly controlled in terms of intensity, wavelength or duration, without affecting any important physiological parameters. In addition, photons can be easily manipulated and focused to achieve precisely localized stimulation. To take full advantage of this spatial property, a concentration of photoresponsive molecules at defined locations is necessary for the consistent release of the target compound. Only a few examples of the functionalization of a nanoparticle surface [10] or the entrapment of photodonors into porous, non-functional scaffolds such as mesoporous silica [11] have been reported. Aside from other macromolecular scaffolds [12] , porous coordination polymers (PCPs) [13] , [14] , [15] , [16] , [17] , [18] , [19] , [20] represent a distinct three-dimensional (3D) framework, assembled from metal ions or clusters and functional organic ligands as building units. Designing appropriate NO photodonor ligands would advantageously render the framework itself photoactive, whereas the loading of NO donors into pores is no longer essential, and potentially toxic photoadducts remain chemically bound to the framework. The ligands are thereby concentrated in a restricted space that exhibits high light-harvesting and NO-reservoir capacities. Moreover, the voids inherent in the framework can offer spatial segregation between the donors, thus preventing the aggregation-induced quenching of reactive excited species [21] , [22] . In line with the strategy to apply PCPs in the biomedical field, relying on the accommodation and subsequent release of drug molecules from the pores [19] , PCP-based NO-releasing materials have been developed based on reversible chemical interactions between NO and accessible open metal sites in the framework [23] , [24] . Recently, by taking advantage of the PCPs hybrid nature, functional ligands were post-synthetically modified into N -diazeniumdiolate donors [25] , [26] . However, in each of these examples the coordination frameworks spontaneously release drug molecules or NO in physiological conditions and the delivery process cannot be initiated or interrupted at a specific time. We propose a new approach for developing on-demand NO delivery platforms based on photoactive PCPs. The assembly of nitro-containing imidazolate ligands, which have low photoreactivity, into well-defined crystalline coordination frameworks leads to a drastic increase in photoreactivity, and the resulting materials can efficiently release NO, only on light irradiation. The applicability of these frameworks for localized cellular delivery is investigated by developing hybrid substrates in which microcrystals of photoactive PCPs are embedded into a biocompatible and gas-permeable polymer matrix to allow cellular adhesion. Two-photon laser scanning confocal microscopy experiments allows for chemical modulation of the cellular microenvironment through the spatiotemporally controlled release of NO. The biological relevance of the delivered NO is demonstrated by a transient increase in the intracellular calcium ion concentration in locally stimulated cells following activation of the NO-sensitive membrane protein. Synthesis and characterization of NO frameworks The development of photoactive PCPs [27] , [28] , [29] , [30] is one of the powerful strategies towards on-demand control of porous properties. However, this approach has never been applied to photoinduced release of biologically relevant molecules. Inspired by NO photodonors based on nitroaromatic compounds, which undergo photoinduced nitro-to-nitrite rearrangement and subsequent bond cleavage to yield NO radicals [31] , [32] , we selected imidazole-based ligands, 2-nitroimidazole (2nIm) and 5-methyl-4-nitroimidazole (mnIm), which are suitable for constructing robust and versatile zeolitic imidazolate frameworks (ZIFs) [33] , [34] , [35] . The solvothermal reaction of zinc nitrate with 2nIm or mnIm in dimethylformamide (DMF) yielded single crystals of [Zn(2nIm) 2 ] n (NOF-1) or [Zn(mnIm) 2 ] n (NOF-2), respectively (NOF, NO framework). Alternatively, homogeneous microcrystalline powders of NOF-1 and NOF-2 were synthesized in a water/DMF mixture at room temperature in the presence of a sodium formate modulator, which induced faster nucleation by ligand deprotonation ( Supplementary Fig. S1 ) [36] . Single-crystal X-ray diffraction (XRD) measurements of both NOF-1 and NOF-2 ( Supplementary Data 1 and 2 ) revealed that the imidazolate ligands bound the zinc ions with a tetrahedral coordination geometry, resulting in the formation of 3D porous coordination frameworks with sodalite (sod) topology. NOF-1 crystallizes as cubic crystal system, I -43 m , which creates a perfectly truncated octahedral sodalite cage ( Fig. 1a ), whereas in NOF-2 the trigonal crystal system, R -3 m , exhibits an elongated sodalite cage along the c axis ( Fig. 1b ). Twelve nitro functionalities are exposed in each sodalite cage without significant interaction with neighbouring atoms ( Supplementary Fig. S2 ). The powder XRD measurements, together with the single-crystal XRD measurements, unambiguously confirmed that NOF-1 and NOF-2 are isostructural to the previously reported ZIF compounds, [Co(2nIm) 2 ] n (ref. 37 ) and [Zn(bIm)] n (ref. 38 ), respectively (bIm, benzimidazole; Fig. 1c and Supplementary Tables S1 and S2 ). 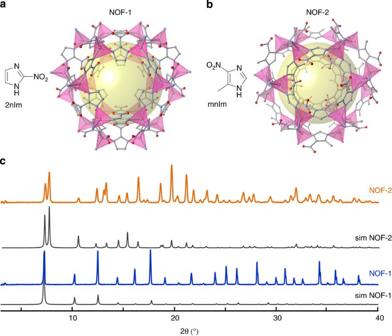Figure 1: Representation of the NO-releasing frameworks. (a,b) The nitro-containing imidazole ligands 2nIm and mnIm were independently reacted in the presence of zinc cations to form the porous sodalite zeolite imidazolate frameworks NOF-1 and NOF-2. (c) The powder XRD peaks of the NOF-1 and NOF-2 match the simulation patterns obtained from the single crystal diffraction data. Figure 1: Representation of the NO-releasing frameworks. ( a , b ) The nitro-containing imidazole ligands 2nIm and mnIm were independently reacted in the presence of zinc cations to form the porous sodalite zeolite imidazolate frameworks NOF-1 and NOF-2. ( c ) The powder XRD peaks of the NOF-1 and NOF-2 match the simulation patterns obtained from the single crystal diffraction data. Full size image To characterize the optical properties of the PCP frameworks, the solid-state ultraviolet–visible absorption spectra of NOF-1, NOF-2, [Co(2nIm) 2 ] n and the imidazole ligands, 2nIm and mnIm, were recorded ( Fig. 2 ). Both ligands present broad and intense absorption bands in the 260–430 nm range, assigned to the n − π * and π − π * transitions of the aromatic nitro functionalities. The similarity between the NOF-1 and 2nIm absorption spectra ( λ max =375 nm) indicates that the electronic environment of the ligand remains essentially unaffected on formation of the crystalline coordination framework; the Zn(II) ions do not become electronically involved in either the ground-state behaviour or the excited-state decay of their coordinating nitrogen-based ligands [39] . The situation is different for [Co(2nIm) 2 ] n , the cobalt analogue of NOF-1; a slightly broadened and bathochromically shifted ultraviolet absorption band and new absorption bands appear in the visible region from 450 to 650 nm ( λ max =550 nm), which can be assigned to the spin-allowed d – d transitions ( 4 A 2 (F)→ 4 T 2 (P)) of the Co(II) centres in a tetrahedral coordination environment [40] . In turn, NOF-2 presents a redshifted absorption maximum ( λ max =450 nm) with respect to mnIm ( λ max =410 nm), reflecting a more planar orientation of the nitro groups in the framework, thereby leading to an increase in electronic delocalization in the aromatic imidazole ring [41] . 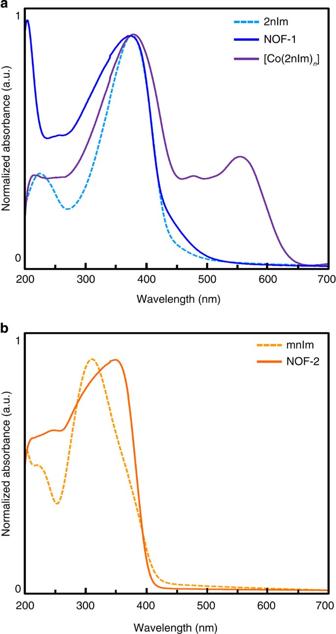Figure 2: UV-Vis diffuse-reflectance spectra of NOF powders and their ligands. (a) The characteristic absorption band assigned to the transition located on the nitro functionality in 2nIm remains unaffected upon the coordination of Zn(II) in NOF-1. As anticipated, [Co(2nIm)2]ngives rise to additional absorption bands in the visible region, which are characteristic of Co(II) in a tetrahedral coordination environment. (b) A bathochromic shift in the absorption band is observed in NOF-2, on the coordination of zinc, which suggests enhancedπ-conjugation in the nitroaromatic ligand. Figure 2: UV-Vis diffuse-reflectance spectra of NOF powders and their ligands. ( a ) The characteristic absorption band assigned to the transition located on the nitro functionality in 2nIm remains unaffected upon the coordination of Zn(II) in NOF-1. As anticipated, [Co(2nIm) 2 ] n gives rise to additional absorption bands in the visible region, which are characteristic of Co(II) in a tetrahedral coordination environment. ( b ) A bathochromic shift in the absorption band is observed in NOF-2, on the coordination of zinc, which suggests enhanced π -conjugation in the nitroaromatic ligand. Full size image Light-induced NO release The NO-releasing properties of NOF-1 and NOF-2 under light irradiation (300-W Xenon lamp, 7.5 mW cm −2 ) were probed using the NO-selective ozone-chemiluminescence technique ( Fig. 3a ). First, the 2nIm and mnIm ligands presented low photoreactivity and produced only limited quantities of NO after 3 h of sustained illumination (release yield=1.4% and 5.9% for 2nIm and mnIm, respectively, based on the conversion of nitro groups to NO). However, when these ligands were organized into crystalline frameworks, their photoreactivity exhibited an increase greater than an order of magnitude under the same illumination conditions; NOF-1 and NOF-2 released 3.4 and 2.9 μmol mg −1 of NO, corresponding to a conversion yield of 50% and 46%, respectively. 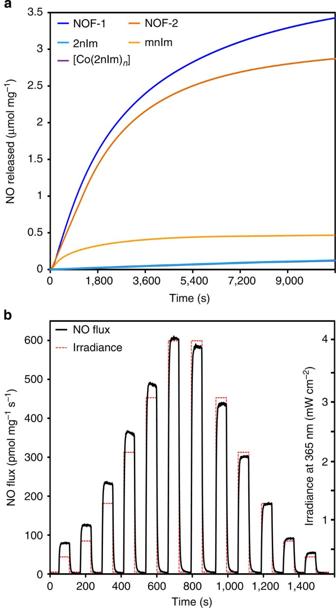Figure 3: Photoinduced NO-releasing properties. (a) The photoreactivity of the ligands 2nIm and mnIm was drastically enhanced on the formation of the PCPs NOF-1 and NOF-2. The [Co(2nIm)2]ndid not release a significant quantity of NO, presumably due to low-energy-lying transitions localized on the Co(II) centre and affording the efficient deactivation of the excited states. (b) The NO flux produced upon the photoactivation of NOF-1 can be tuned by varying the intensity of the light source. When the irradiation is interrupted, the NO production is instantly terminated and no leakage is observed in the dark state. Figure 3: Photoinduced NO-releasing properties. ( a ) The photoreactivity of the ligands 2nIm and mnIm was drastically enhanced on the formation of the PCPs NOF-1 and NOF-2. The [Co(2nIm) 2 ] n did not release a significant quantity of NO, presumably due to low-energy-lying transitions localized on the Co(II) centre and affording the efficient deactivation of the excited states. ( b ) The NO flux produced upon the photoactivation of NOF-1 can be tuned by varying the intensity of the light source. When the irradiation is interrupted, the NO production is instantly terminated and no leakage is observed in the dark state. Full size image Although the values are comparable, NOF-1 exhibits a moderately superior NO-releasing efficiency to that of NOF-2 (under a 300- to 600-nm light irradiation), which can be explained by the improved light-absorption capacity of NOF-1 ( Fig. 2 ) due to the nitro substitution position on the imidazole ring; NOF-1 demonstrates significant absorption tailing in the range of 400–500 nm. The absorption spectra imply that the increase in the photoreactivity of the framework compounds over that of their respective ligands cannot be assigned to the perturbation of the electronic environment of the ligands upon Zn(II) coordination. As with the solid-state luminescence quenching effect observed in most fluorescent organic compounds, the inefficiency with which both mnIm and nIm release NO from their aggregated form on light irradiation can be explained by intermolecular interactions (favouring the formation of excimers) that provide efficient non-reactive deactivation pathways for the excited states [42] . In contrast, as observed from their crystal structures, the porous frameworks of NOF-1 and NOF-2 provide sufficient spatial segregation to prevent intermolecular ligand interactions and thus an excited-state deactivation [21] , [22] . The lack of NO production by the methylimidazolate-based reference material, [Zn(MeIm) 2 ] n (ZIF-8) [36] , supports the photochemical involvement of the nitro groups in the formation of NO ( Supplementary Fig. S3 ). As confirmed by gas chromatography-mass spectrometry (GCMS) analysis, NO was the only nitrogen oxide species released after the irradiation of NOF-1 ( Supplementary Fig. S4 ). Interestingly, the cobalt framework [Co(2nIm) 2 ] n failed to release significant quantities of NO (2%) compared with NOF-1 ( Fig. 2 ). As observed in the ultraviolet–visible spectrum, the ligand field and other low-energy states present on the cobalt centre can deactivate the excited states localized on the functional ligands and disfavour the photochemical deactivation pathway. These observations underline the importance of the choice in metal ion to the construction of efficient photoactive frameworks. Furthermore, we obtained a two-dimensional non-porous framework, referred to as NOF-3, assembled from the 2nIm ligand and Zn(II) ions, [Zn(2nIm)(HCOO)] n , by modifying the reaction conditions. Compared with NOF-1, the amount of NO released upon similar illumination was significantly reduced in the dense framework (1.2 μmol mg −1 after 3 h; Supplementary Figs. S5–S9 ). This observation supports our design strategy through which efficient NO-releasing properties can be achieved by constructing suitable porous frameworks from NO photodonor building blocks. In addition to high releasing efficiency, spatiotemporal control over the produced NO flux is important to NO delivery systems. We investigated the illumination of NOF-1 under variable light power ( Fig. 3b and Supplementary Fig. S10 ). NO is released instantly on photoactivation and the NO flux can be easily tuned by both the irradiation intensity and the amount of irradiated material. As anticipated, the production of NO is immediately interrupted when the irradiation ceases and its concentration quickly drops to trace levels. NOF powders did not present any significant decrease in crystallinity or in NO release after 8 months of storage under ambient conditions ( Supplementary Fig. S11 ). In addition, the lack of significant NO release when heated up to 200 °C, confirmed the thermal stability of NOF powders and that NO is produced exclusively through a photochemical process ( Supplementary Fig. S12 ). Spatiotemporally controlled release in cell media To render our compounds biologically applicable, we prepared NOF-based substrates suitable for cell cultures and microscopic imaging ( Fig. 4a ); NOF-1 microcrystals were first spin-cast on a glass-bottomed dish. Next, a biocompatible polydimethylsiloxane (PDMS) layer was spin-coated on top to embed the crystals completely in a polymer matrix with a reproducible thickness (20±5 μm). Notably, the crystal distribution on the glass surface did not seem to be altered by the spin-coating process and the NOF crystals remained on the bottom part of the polymer layer ( Fig. 4b and Supplementary Fig. S13 ). As confirmed by irradiation experiments, the thin PDMS layer allowed for the diffusion of released NO ( Supplementary Fig. S14 ). Although moderately slowing the release kinetics, the total quantity of NO released remained comparable to that of the uncoated material. In addition, the fine tuning of the light intensity allowed a sustained and adjustable flux of NO for 2 h (250 pmol mg −1 s −1 for 1 h, then 350 pmol mg −1 s −1 for another hour by using increased light power; Supplementary Fig. S15 ). 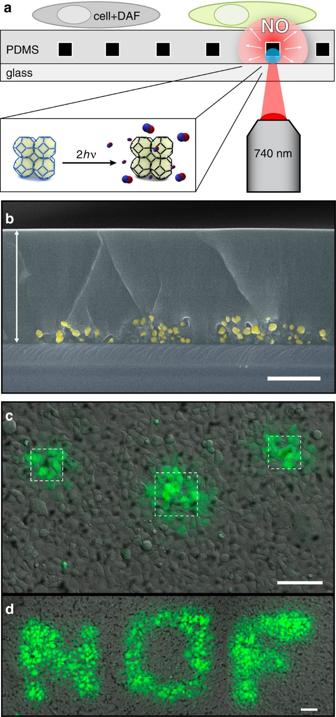Figure 4: Spatiotemporally controlled release of NO. (a) Schematic illustration of the localized cell-stimulation platform. The PDMS-embedded NOF-1 crystals are locally photoactivated by two-photon near-infrared laser irradiation. The generated NO diffuses through the PDMS layer and reacts with an intracellular NO fluorescent indicator, DAF-FM. (b) Cross-section scanning electron microscopy image of NOF-1/PDMS substrate. The white arrow highlights the homogeneous PDMS layer. NOF-1 crystals (yellow) are localized on the bottom part of the substrate, ensuring their isolation from the cellular medium (scale bar, 10 μm). (c) Confocal microscopy images of NOF-1-embedded substrates cultured with HEK293 cells introduced via DAF-FM. The selective photoactivation of the NOF-1 crystals (white squares) induced a fluorescent response in the surrounding cells, highlighting the localized NO delivery and uptake (scale bar, 100 μm). (d) Further demonstration of spatiotemporal control by writing ‘NOF’ upon activation of the selected regions (scale bar, 100 μm). Figure 4: Spatiotemporally controlled release of NO. ( a ) Schematic illustration of the localized cell-stimulation platform. The PDMS-embedded NOF-1 crystals are locally photoactivated by two-photon near-infrared laser irradiation. The generated NO diffuses through the PDMS layer and reacts with an intracellular NO fluorescent indicator, DAF-FM. ( b ) Cross-section scanning electron microscopy image of NOF-1/PDMS substrate. The white arrow highlights the homogeneous PDMS layer. NOF-1 crystals (yellow) are localized on the bottom part of the substrate, ensuring their isolation from the cellular medium (scale bar, 10 μm). ( c ) Confocal microscopy images of NOF-1-embedded substrates cultured with HEK293 cells introduced via DAF-FM. The selective photoactivation of the NOF-1 crystals (white squares) induced a fluorescent response in the surrounding cells, highlighting the localized NO delivery and uptake (scale bar, 100 μm). ( d ) Further demonstration of spatiotemporal control by writing ‘NOF’ upon activation of the selected regions (scale bar, 100 μm). Full size image To deliver NO in a localized cellular environment, we utilized the high spatiotemporal resolution of confocal laser scanning microscopy, which allowed for precise and localized photoactivation of the NOF-1/PDMS substrates and subsequent rapid observation of the cellular response. As the absorption of our material was essentially in the ultraviolet region, we used a near-infrared two-photon laser to photoactivate NOF-1, thus greatly reducing the risk of photodamaging the cells with harmful ultraviolet irradiation while effectively inducing the NO release. The sterilized NOF-1/PDMS were coated with Matrigel to facilitate cell adhesion and growth, and then human embryonic kidney 293 (HEK293) cells were cultured on this substrate ( Supplementary Fig. S16 ). Compared with pristine PDMS substrates, the presence of NOF-1 in the polymer layer did not induce any notable cytotoxicity ( Supplementary Fig. S17 ). We predicted that the high spatial resolution of the two-photon confocal laser would allow for the selective activation of any crystals chosen to enable localized NO delivery to the surrounding cells. Before the activation experiments, DAF-FM DA (4-amino-5-methylamino-2′,7′-difluorofluorescein diacetate) [43] , a cell-permeable NO fluorescent indicator, was introduced into the HEK293 cells. As shown in Fig. 4c,d , the rapid photoactivation of a selected region containing NOF-1 crystals quickly induced an increase in the fluorescence of the surrounding HEK293 cells. Within seconds, the NO generated from NOF-1 was able to diffuse through the PDMS layer to the cellular membrane and further reacted with the NO indicator to form a fluorescent adduct. These results clearly suggest a high degree of spatiotemporal control over the NO delivery using a simple, reproducible and extremely fast two-photon photoactivation process. As control experiments, [Zn(MeIm) 2 ] n microcrystals (lacking nitro functions) and an area of the PDMS substrate without any microcrystals were irradiated under identical photoactivation conditions. The irradiation did not induce any increase in the intracellular DAF-FM fluorescence in the surrounding cells ( Supplementary Fig. S18 ). Having demonstrated rapid NO delivery into cells with spatiotemporal precision, we aimed to probe the biological relevance of the NO released from photoactive PCP by observing an NO-activated cellular response. Calcium ions (Ca 2+ ) have a key role in regulating many physiological processes in mammalian cells, including neurotransmission, muscle contraction, proliferation, fertilization and apoptosis [44] . In this context, we targeted an NO-sensing transmembrane channel protein, transient receptor potential channel 5 (TRPC5), which undergoes a conformational change in the presence of NO, allowing for an influx of extracellular Ca 2+ ion into the cells ( Supplementary Fig. S19 ) [45] . We investigated whether the photoactivated release of NO from NOF-1/PDMS substrates was able to change the intracellular calcium concentration, [Ca 2+ ] i , in HEK293 cells genetically modified to express the TRPC5 transmembrane channel (HEK293-TRPC5). After introducing a fluorescent Ca 2+ indicator (Fluo-4) into the cells, we monitored the changes in [Ca 2+ ] i in the native HEK293 and the modified HEK293-TRPC5 cells after the two-photon photoactivation of NOF-1. As depicted in Fig. 5 , although the NO delivered to the control native HEK293 cells did not affect [Ca 2+ ] i , a rapid [Ca 2+ ] i response in the surrounding HEK293-TRPC5 cells was observed upon photoactivation of comparable quantities of NOF-1 crystals ( Supplementary Figs S20 and S21 and Supplementary Movies 1 and 2 ). These results indicate that NO released from the photoactivated PCP reacted with the TRPC5 channel on the cell membrane and triggered its opening. Note that the fluorescence intensity of Fluo-4 in the cells peaked after a few to several tens of seconds and, in most cases, decreased towards its initial level within a few minutes. This observation is in accordance with the transient nature of the NO delivery provided by the NOF-1 substrate with the rapid initiation and termination of its NO release. As previously observed in the NO-monitoring experiments conducted using DAF-FM, the irradiation of substrates incorporating [Zn(MeIm) 2 ] n did not alter [Ca 2+ ] i in the HEK293 or HEK293-TRPC5 cells ( Supplementary Fig. S22 ). 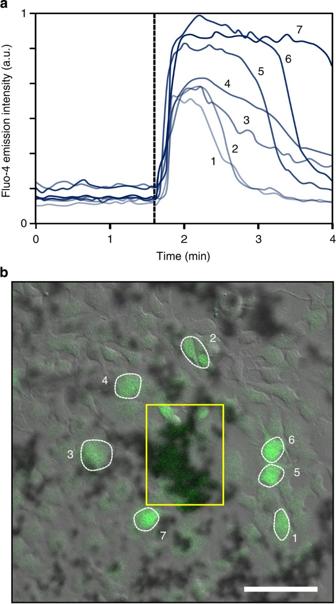Figure 5: Downstream signalling triggered by NO delivery. (a) Emission intensity profile of Fluo-4 in the HEK293-TRPC5 cells, accounting for the intracellular calcium ion concentration, [Ca2+]i, before and after the photoactivation of NOF-1 (dashed line indicates initiation). The curves refer to the fluorescence of the circled cells inFig. 5b. (b) Confocal microscopy image obtained after the irradiation of NOF-1 crystals (yellow rectangle) showing increased fluorescence of Fluo-4 in the HEK293-TRPC5 cells surrounding the photoactivation area (scale bar, 100 μm). Figure 5: Downstream signalling triggered by NO delivery. ( a ) Emission intensity profile of Fluo-4 in the HEK293-TRPC5 cells, accounting for the intracellular calcium ion concentration, [Ca 2+ ] i , before and after the photoactivation of NOF-1 (dashed line indicates initiation). The curves refer to the fluorescence of the circled cells in Fig. 5b . ( b ) Confocal microscopy image obtained after the irradiation of NOF-1 crystals (yellow rectangle) showing increased fluorescence of Fluo-4 in the HEK293-TRPC5 cells surrounding the photoactivation area (scale bar, 100 μm). Full size image Light-induced NO release from macromolecular assemblies or solid-state materials has been achieved essentially by immobilizing NO photodonors on the surface of nanoparticles [10] or accommodating them in host scaffolds such as mesoporous silica [11] . Here we propose a different approach where the NO photodonors themselves are the building units, organized into 3D porous coordination structures. The spatial segregation of the functional components in porous frameworks, with electronically non-involved metal centres, allowed a drastic increase in the photo reactivity by preventing the quenching of the reactive excited states. This advantageous accumulation of photoactive donors in PCP architectures lead to efficient and tunable light-induced NO release and places NOF materials (3.4 μmol mg −1 for NOF-1) above the most efficient, controllable solid-state NO-delivery scaffolds (1.3 μmol mg −1 for nitrosothiol-modified silica xerogels) [12] . Notably, their excellent stability under ambient conditions avoids the need of cautious handling or storage (as required with light-sensitive metal-nitrosyls or thermally unstable nitrosothiols). This work suggests a great potential of PCPs for controllable light-induced release of biologically relevant molecules. To take advantage of the concentration of photodonor ligands in the PCP structure, we prepared a new NO cell-stimulation platform by immobilizing the NOF-1 microcrystals in a permeable and biocompatible polymer layer, and we confirmed that the irradiation of NOF-1/PDMS could generate relevant and sustained flux of gaseous NO, which easily diffused through the polymer layer. A high degree of spatiotemporal control over the NO delivery was achieved using harmless near-infrared two-photon laser activation and allowed for a precisely localized stimulation of cells surrounding the photoactivated crystals. We have further demonstrated the biological relevance of this exogenous NO delivery by observing the subsequent cellular response, that is, a transient increase in the intracellular calcium concentration, triggered by the conformational change in a NO-sensitive transmembrane channel. Aside from the potential therapeutic applications, we believe this approach could provide valuable fundamental understanding of the physiological and pathophysiological roles of NO, particularly the functions of NO in brain circuitry in which the spatiotemporal generation of stimulating molecules in subcellular domains is desired. Preparation of single crystals of NOF-1 The 2-nIm (113 mg, 1.0 mmol) and Zn(NO 3 ) 2 ·6H 2 O (149 mg, 0.5 mmol) were dissolved in DMF (5 ml) in a sealed microwave vial. The solution was heated to 100 °C via microwave irradiation for 1 h. Individual yellow crystals appeared on the glass. The yield could be increased by heating the mixture in a 100 °C oven for 24 h. Preparation of single crystals of NOF-2 MnIm (25 mg, 0.20 mmol) and Zn(NO 3 ) 2 ·6H 2 O (21 mg, 0.07 mmol) were dissolved in DMF (3 ml) in a glass tube. The solution was heated in a 100 °C electric oven. After 48 h, light-yellow single crystals appeared on the glass. Preparation of single crystals of NOF-3 2-Nitroimidazole (23 mg, 0.20 mmol) and Zn(NO 3 ) 2 ·6H 2 O (30 mg, 0.10 mmol) were dissolved in a DMF-H 2 O mixture (v/v 1/1, 1 ml) in a glass tube and heated in an oil bath at 100 °C for 36 h to afford pale yellow plate-like single crystals. Preparation of microcrystalline NOF-1 and NOF-2 powders 2-nIm (113 mg, 1.0 mmol) or mnIm (127 mg, 1.0 mmol) and sodium formate (136 mg, 2.0 mmol) were dissolved in a DMF/H 2 O (v/v, 10/1) mixture (5 ml). A solution of Zn(NO 3 ) 2 ·6H 2 O (149 mg, 0.5 mmol) in H 2 O (5 ml) was later added, and the reaction mixture was stirred vigorously at room temperature. The reaction mixture became cloudy within a few minutes after adding the zinc solution. After 18 h, the precipitate was centrifuged and washed with water (2 × 15 ml) and DMF (3 × 15 ml) to yield NOF-1 (68 mg, 27%) as a pale yellow powder or NOF-2 (35 mg, 13%) as a white powder. A solvent-exchange procedure was performed by immersing the powders successively in fresh methanol (4 × 15 ml over 48 h). The compounds were then heated under reduced pressure (80 °C, 10 mbar) for 18 h. Anal. calculated for NOF-1, C 6 H 4 N 6 O 4 Zn=Zn(2nIm) 2 : C, 24.89; H, 1.39; N, 29.03; found: C, 24.77; H, 1.61; N, 28.08. Anal. calculated for NOF-2, C 11 H 15 N 7 O 5 Zn=Zn(mnIm) 2 . (DMF): C, 33.82; H, 3.87; N, 25.10; found: C, 33.27; H, 3.57; N, 25.20. Preparation of microcrystalline NOF-3 powder 2-Nitroimidazole (113 mg, 1.00 mmol) and Zn(NO 3 ) 2 ·6H 2 O (297 mg, 1.00 mmol) were dissolved in DMF (10 ml) by microwave irradiation at 100 °C for 6 h. The resulting product was washed with DMF (3 × ) to afford a pale yellow powder (200 mg, 90%). Anal. calculated for C 4 H 3 N 3 O 4 Zn=Zn(2nIm)(HCO 2 ): C, 21.59; H, 1.36; N, 18.89; found: C, 21.35; H, 1.37; N, 18.67. Preparation of [Co(2nIm)2] n (ZIF-65) 2-Nitroimidazole (90 mg, 0.80 mmol) and Co(NO 3 ) 2 ·6H 2 O (120 mg, 0.40 mmol) were dissolved in DMF (4 ml) in a glass vial. The solution was heated in an electric oven for 6 h at 120 °C and then cooled down to room temperature within 12 h. Block crystal of [Co(2nIm)2] n formed on the glass vial. The mother liquor was quickly filtered while hot. After few minutes, a microcrystalline powder of ZIF-65 precipitated at room temperature. The purple powder was centrifuged and washed with DMF (3 × ). Anal. calculated for C 9 H 13 CoN 7 O 6 =Co(2nIm) 2 ·(DMF)(H 2 O): C, 28.89; H, 3.50; N, 26.20; found: C, 28.81; H, 3.46; N, 25.58. Crystal structure determination Single crystals of NOF-1, NOF-2 or NOF-3 were placed on a MicroLoops with Paraton-N (Hampton Research) and mounted on a Rigaku AFC10 diffractometer with Rigaku Saturn Kappa CCD system equipped with a MicroMax-007 HF/VariMax rotating-anode X-ray generator with confocal monochromatized MoKα ( γ =0.71069 Å) radiation. The crystal structures were solved by a direct method and refined by full-matrix least-squares refinement using the SHELXL-97 ( Supplementary Tables S1–S3 and Supplementary Data 1 , 2 , 3 ). All non-hydrogen atoms were refined anisotropically with hydrogen atoms generated as spheres riding the coordinates of their parent atoms. Solvent molecules were removed by SQUEEZE procedure. Powder X-ray diffraction Measurements were performed with a Bruker D8 operating with Cu Kα radiation ( λ =1.54 Å) with a 40-kV beam voltage and 40-mA current. Field-emission scanning electron microscopy Observations were performed with a JEOL Model JSM-7001F4 scanning electron microscopy system operating at 15.0 kV. The samples were deposited on carbon tape and coated with osmium before measurement. Gas chromatography mass spectroscopy Analyses were performed with a Shimadzu GCMS-QP5050A, using a ZB-1 (polymethylsyloxane) column (60 m × 0.32 mm and 5.0 μm thickness). The column temperature was 40 °C and the temperature of injection was 200 °C with helium gas carrier (pressure, 80 kPa; flow rate, 2 ml min −1 ). Mass spectrometer was operated at 200 °C with an ionization voltage of 70 eV and ionization current of 60 mA. Light-induced NO release Methanol suspensions of NOF microcrystals (~2 mg ml −1 ) were repeatedly spin-cast (2,000 r.p.m.) on a 22 × 22-mm cover slip and activated under reduced pressure for 3 h (10 mbar, 85 °C). The weight of the deposited material was accurately determined using a precision scale (typical weights, 80–120 μg). The samples were placed in a custom-made cell and irradiated with a 300-W Xenon lamp (Asahi Spectra Max-303 equipped with a 300- to 600-nm ultraviolet–visible module and × 1.0 collimator lens). The incident light power at 365 nm was measured using an Ushio UIT-201 intensity meter. The NO release measurements were performed using a Sievers NOA 280i chemiluminescence NO analyser. The instrument was calibrated by passing air through a zero filter (Sievers, <1 ppb NO) and 640 ppb NO gas. The nitrogen carrier gas flow rate was set to 200 ml min −1 with a cell pressure of 8.5 Torr and an oxygen pressure of 6.1 psig. Substrate preparation A methanolic suspension of NOF-1 was repeatedly spin-cast (2,000 r.p.m.) onto a glass-bottomed culture dish. The crystals were embedded in a PDMS layer by spin-coating a pre-polymer/curing agent mixture (w/w, 10/1, Sylgard 184) at 3,000 r.p.m. for 1 min to allow the formation of a reproducible 15- to 20-μm-thick polymer layer (determined via laser scanning confocal microscopy and scanning electron microscopy). The substrate was heated at 80 °C under reduced pressure for an additional 18 h. Cell culture The HEK293 and HEK293-TRPC5 cells were cultured in medium consisting of DMEM supplemented with 10% (v/v) fetal bovine serum and 1% (v/v) penicillin/streptomycin in a humidified incubator (37 °C, 5% CO 2 ). The medium was changed every 2–3 days. The cells were passaged with trypsin-EDTA solutions. For the HEK293-TRPC5 cells, 100 μg ml −1 G418 was added to the culture medium for their selection. Cell culture on an NOF-1/PDMS substrate Before cell culture, a NOF-1/PDMS substrate was sterilized using 70% ethanol and coated with Matrigel (BD Bioscience, USA; certified for human embryonic stem cell culture) that had been diluted with DMEM/Ham F12 medium to facilitate cell adhesion and growth at 4 °C overnight. The substrate was then rinsed with cell culture medium twice to remove any excess Matrigel. The trypsinized HEK293 or HEK293-TRPC5 cells (1 × 10 5 cells) were introduced onto a substrate and cultured until the experiments were performed. For the HEK293-TRPC5 cells, a culture medium with 100 μg ml −1 G418 was used, but replaced with fresh culture medium without G418 1 day before the experiments. Fluorescence imaging A Fluo-4 (molecular probe; 1 μM) or DAF-FM (molecular probe; 5 μM) was introduced into the cells in culture medium 30 min before the imaging experiments. After the incubation period, the cells were quickly rinsed once with PBS and imaged in Tyrode’s solution (129 mM NaCl, 5 mM KCl, 2 mM CaCl 2 , 1 mM MgCl 2 , 30 mM glucose, 25 mM HEPES and 0.01 mM glycine). Laser scanning confocal microscopy experiments All fluorescent images used for cell imaging were acquired on an Axio Observer Z1 mounted with a live-cell imaging chamber, a motorized XY-stage, a Plan-Apochromat 20 × /0.80 objective (LSM780, Zeiss) and a Chameleon VISION II (680–1,080 nm) two-photon laser (Coherent Inc.). The imaging parameters for the Fluo-4 and DAF-FM (excitation at 488 nm, emission at 493/545 nm) were determined based on information provided by the manufacturer. Apoptosis assay Cell apoptosis were detected with Annexin V apoptosis detection kit APC (eBioscience). Briefly, cells were washed twice with PBS and collected with 0.25% trypsin in PBS (Invitrogen). Cells were suspended in cell culture medium and placed in 15-ml tubes. After centrifugation at 1,000 r.p.m. for 5 min, the supernatant was removed. Cells were washed with PBS and binding buffer (eBioscience), and then counted. For staining, cells were diluted to 5 × 106 cells ml −1 in binding buffer. Annexin V labelled with allophycocyanin were added and incubated at room temperature for 15 min. Cells were centrifuged at 1,000 r.p.m. for 5 min and then washed with binding buffer. Cells were centrifuged and resuspended in binding buffer to which propidium iodide was added. Labelled cells were analysed with a FACS Canto II (BD Biosciences). Accession codes: The X-ray crystallographic coordinates and structure factors for NOF-1, NOF-2 and NOF-3 have been deposited at the Cambridge Crystallographic Data Centre (CCDC) under accession codes 917446 to 917448, respectively. These data can be obtained free of charge from the Cambridge Crystallographic Data Centre via http://www.ccdc.cam.ac.uk/data_request/cif . How to cite this article: Diring, S. et al . Localized cell stimulation by nitric oxide using a photoactive porous coordination polymer platform. Nat. Commun. 4:2684 doi: 10.1038/ncomms3684 (2013).